Complete tomography of a high-fidelity solid-state entangled spin–photon qubit pair Entanglement between stationary quantum memories and photonic qubits is crucial for future quantum communication networks. Although high-fidelity spin–photon entanglement was demonstrated in well-isolated atomic and ionic systems, in the solid-state, where massively parallel, scalable networks are most realistically conceivable, entanglement fidelities are typically limited due to intrinsic environmental interactions. Distilling high-fidelity entangled pairs from lower-fidelity precursors can act as a remedy, but the required overhead scales unfavourably with the initial entanglement fidelity. With spin–photon entanglement as a crucial building block for entangling quantum network nodes, obtaining high-fidelity entangled pairs becomes imperative for practical realization of such networks. Here we report the first results of complete state tomography of a solid-state spin–photon-polarization-entangled qubit pair, using a single electron-charged indium arsenide quantum dot. We demonstrate record-high fidelity in the solid-state of well over 90%, and the first (99.9%-confidence) achievement of a fidelity that will unambiguously allow for entanglement distribution in solid-state quantum repeater networks. Over the past two decades, entanglement between remote quantum systems has had a key role within the nascent field of quantum information [1] , [2] , particularly so in quantum communication. Not only can entangled states be used for the generation of unconditionally secure cryptographic keys [1] ; an entangled pair of quantum systems can be used as a resource to teleport quantum states [3] . In addition, entanglement is self-propagating: under certain, well-understood conditions, two pairs of entangled states can be used to generate a new pair, by performing joint Bell-state measurements [4] on one state of each pair—in a process known as entanglement swapping [5] . This process can be used to generate remote entanglement between stationary quantum memories that never interacted, by performing a probabilistic, partial Bell-state measurement through two-photon interference of the photonic part of two entangled pairs, each consisting of the quantum memory and a photonic qubit [6] . The resulting state from the post-selective process is one in which the quantum memories are entangled. Using such a scheme, in combination with local Bell-state measurements, gives rise to a quantum relay, where entanglement propagates along a chain of nodes [7] , [8] . Quantum repeaters, built in this way, are crucial for developing long-distance quantum communication networks [9] , [10] , [11] . Such schemes rely on the generation and/or existence of high-fidelity entangled states and intermediate Bell-state measurement; as otherwise errors would propagate and quickly make the end states fully mixed (classical). Perfect entanglement and Bell-state measurement, of course, do not exist in practice. The canonical solution to this problem, entanglement purification [12] , [13] , [14] , consists of the distillation of high-fidelity entangled states out of lower-fidelity precursors. The combination of entanglement purification with a quantum relay of remotely entangled quantum memories is the essence of a quantum repeater [7] , [8] , where many parallel, sacrificial links are used to generate remote entanglement in a nested protocol that combines entanglement purification with entanglement swapping. The number of parallel links required depends, in a nonlinear way, on the initial fidelity of the entangled pairs [8] , and deteriorates rapidly with decreasing initial state fidelity. This immediately leads to a particular conundrum: although high-fidelity entanglement and quantum operations have been demonstrated for well-isolated systems such as trapped ions [15] , [16] , [17] and atoms [10] , [11] , such systems do not lend themselves easily to the sort of large-scale parallelism that would be required to overcome their residual errors. Conversely, in the solid-state, where massive parallelism appears more realistic, the fidelity of quantum memory–photon entanglement in nitrogen-vacancy diamond [18] and optically active quantum dots [19] , [20] , [21] has so far remained rather poor, which would require ever-larger overheads in terms of parallelism to correct for the local imperfections. In this work, we present results from a solid-state spin–photon entanglement setup that we previously [21] used to demonstrate a proof-of-principle, and with which we placed a bound on entanglement fidelity of F >0.8. We have optimized the setup, and now demonstrate, via full state tomography (which has not been previously reported for any solid-state spin–photon experiment at optical frequencies [20] , [21] ), a record-high solid-state spin–photon entanglement fidelity, with levels approaching, or in some cases surpassing, reported ion–photon [15] , [17] and atom–photon [22] , [23] entanglement fidelities. Spin–photon entanglement via optimized quantum erasure We use a single InAs quantum dot electron spin as the stationary qubit [24] , [25] (see Fig. 1a ). A magnetic field in the Voigt geometry (in-plane, perpendicular to the growth direction, B =3T) provides a natural quantization axis, and allows for optical initialization [26] and ultrafast, high-fidelity optical control [25] . In addition, interference between the spontaneous emission decay pathways in the resulting Λ-systems results in entanglement between the spin and the photon [19] , [20] , [21] , see Fig.1b . The large magnetic field results in a Zeeman energy splitting, δω , of 2 π × 17.6 GHz. Conversely, the equivalent frequency difference between the H- and V-polarized branches of the spontaneous emission decay, δω , can result in frequency-which-path information leaking out to the environment [21] , [19] . By mixing a short gating pulse with the single photon in a nonlinear crystal (a periodically poled lithium niobate (PPLN) waveguide [21] , [27] , see Fig. 1c ), we can postselect for the photon’s exact arrival time, with sub-8 ps timing resolution and with negligible background noise. The bandwidth of this detection scheme, about 100 GHz, greatly exceeds the frequency-which-path information of 17.6 GHz; this scheme is therefore inherently incapable of distinguishing the frequency difference, resulting in quantum erasure. As the timing resolution is not infinite, the environment can nevertheless still obtain some partial information, yielding a theoretical fidelity bound of about 95%. The quantum dot manipulation scheme and the system diagram are indicated in Fig. 1d,e . We first initialize the system by a 13-ns optical pumping pulse [25] , [26] . Then, a 100-ps optical π -pulse excites the quantum dot into the -state, after which spontaneous emission results in spin-polarization entanglement. 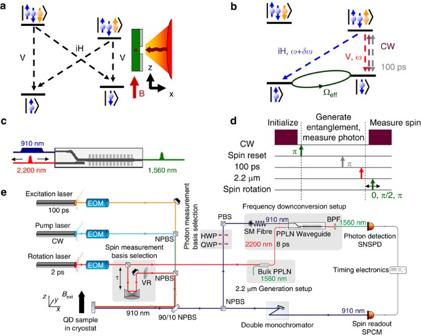Figure 1: Outline and setup of the spin–photon entanglement experiment. (a) Level structure of an electron-doped quantum dot, with the magnetic field in-plane (Voigt geometry, see inset). V and H refer to linear polarizations, either perpendicular to (V) or parallel (H) to the magnetic field. (b) Excitation and manipulation used in the experiment. See text for details. CW: continuous-wave laser, used for spin initialization and read-out. 100 ps: 100 ps laser pulse used for trion excitation.δω: Zeeman energy splitting (2π× 17.6 GHz). Ωeff: effective spin-Rabi frequency of the detuned coherent-spin rotation laser. (c) Schematic overview of the time-resolved conversion process. A few-ps, 2.2-μm gate pulse converts a single 910-nm photon to a 1560-nm photon with picosecond timing resolution in a periodically poled lithium niobate waveguide. The resulting timing resolution acts as a quantum eraser for frequency-which-path information present in the spontaneous emission decay from the Λ-system, permitting high-fidelity spin-polarization entanglement to be measured. (d) Timing and pulse scheme used for generating and verifying spin–photon entanglement. (e) Schematic overview of the experimental apparatus. EOM: electro-optic modulator; VR: variable retarder; H(Q)WP: half-(quarter-)waveplate; (N)PBS: (non-)polarizing beamsplitter; PPLN: periodically poled lithium niobate; QD: quantum dot; SM: single-mode; BPF: bandpass filter. Figure 1: Outline and setup of the spin–photon entanglement experiment. ( a ) Level structure of an electron-doped quantum dot, with the magnetic field in-plane (Voigt geometry, see inset). V and H refer to linear polarizations, either perpendicular to (V) or parallel (H) to the magnetic field. ( b ) Excitation and manipulation used in the experiment. See text for details. CW: continuous-wave laser, used for spin initialization and read-out. 100 ps: 100 ps laser pulse used for trion excitation. δω : Zeeman energy splitting (2 π × 17.6 GHz). Ω eff : effective spin-Rabi frequency of the detuned coherent-spin rotation laser. ( c ) Schematic overview of the time-resolved conversion process. A few-ps, 2.2-μm gate pulse converts a single 910-nm photon to a 1560-nm photon with picosecond timing resolution in a periodically poled lithium niobate waveguide. The resulting timing resolution acts as a quantum eraser for frequency-which-path information present in the spontaneous emission decay from the Λ-system, permitting high-fidelity spin-polarization entanglement to be measured. ( d ) Timing and pulse scheme used for generating and verifying spin–photon entanglement. ( e ) Schematic overview of the experimental apparatus. EOM: electro-optic modulator; VR: variable retarder; H(Q)WP: half-(quarter-)waveplate; (N)PBS: (non-)polarizing beamsplitter; PPLN: periodically poled lithium niobate; QD: quantum dot; SM: single-mode; BPF: bandpass filter. Full size image Complete tomography of the spin–photon entangled qubit pair We perform joint, time-resolved measurements on the polarization state of the photon (polarization analysing stage in Fig. 1e ), and the spin state. The latter can be measured by a combination of a few-picoseconds, high-fidelity, all-optical spin rotation pulse [25] , [28] and another optical pumping pulse to read out the spin in its computational ( , ) basis. Together, this allows us to perform complete state tomography of the entangled spin–photon-polarization qubit pair [29] , [30] , and enables us to compare the experimentally obtained entangled state with the theoretical, ideal spin-polarization entangled state (assuming no errors and perfect frequency quantum erasure—see Supplementary Note 1 ): In quantum state tomography, one aims to reconstruct the density matrix, ρ reconstructed of the experimentally obtained quantum state by means of a set of linearly independent measurements [29] , [30] . This density matrix approaches the theoretical one, ρ ideal = , with the difference vanishing in the limit of arbitrarily small errors in both the generation process and the measurement performed to reconstruct the density matrix. For a two-qubit system, and assuming proper normalization, a minimum of 15 linearly independent measurements is required to reconstruct the density matrix: ρ reconstructed = , where σ i , σ j refer to the Pauli operators of the respective qubits ( σ 0 = I , the identity operator). As the Pauli operators are the generators of quantum mechanical qubit rotations, the coefficients r i , j =Tr[ ρ reconstructed σ i σ j ] are related to the joint measurement of both qubits after applying single qubit rotations on both of them [29] . In particular, the joint measurement is calculated through comparing the coincidence counts between our spin and photon measurement devices, and comparing them to the coincidences obtained in different, uncorrelated events. For our photonic polarization qubit, we measure both in the {H,V} computational basis, and in two rotated bases, by means of our polarization analysing stage: and . For the spin qubit, we change the measurement basis by applying a rotation pulse ( π or π /2) with the appropriate delay to change the rotation axis [25] ; the bases we measure in are: , , . Each coincidence measurement results in a conditional probability, using which the r i , j can be computed. From the 36 potential joint measurement settings resulting from these states, we choose a subset of 16 (15+1), that are linearly independent, which results in a straightforward, direct reconstruction of an initially unnormalized density matrix using the above definition and arithmetic manipulation—see Supplementary Note 2 . Normalization of the density matrix then follows from a simple division by the trace, as suggested by James et al. [30] . The result of this direct reconstruction is indicated in Fig. 2 , where we compare the thus obtained density matrix with the ideal one. The overlap with the ideal state, yields a fidelity of 92.7%. However, due to measurement errors, this density matrix is non-physical (non-positive); in particular, one of the eigenvalues is negative: −0.19. 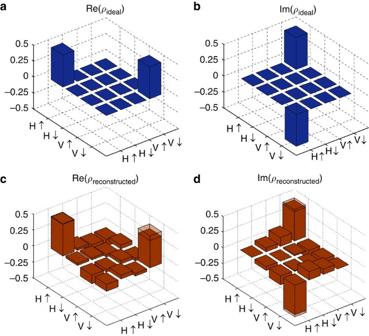Figure 2: Direct density matrix reconstruction. (a) Real part of the density matrix of the ideal spin–photon entangled state,ρideal=. (b) Imaginary part of the density matrix of the ideal spin–photon entangled state,ρideal=. (c) Real part of the reconstructed density matrixρreconstructed, overlayed on the ideal density matrix (shaded box). (d) Imaginary part of the reconstructed density matrixρreconstructed, overlayed on the ideal density matrix (shaded box). Figure 2: Direct density matrix reconstruction. ( a ) Real part of the density matrix of the ideal spin–photon entangled state, ρ ideal = . ( b ) Imaginary part of the density matrix of the ideal spin–photon entangled state, ρ ideal = . ( c ) Real part of the reconstructed density matrix ρ reconstructed , overlayed on the ideal density matrix (shaded box). ( d ) Imaginary part of the reconstructed density matrix ρ reconstructed , overlayed on the ideal density matrix (shaded box). Full size image MLE reconstruction of the spin–photon density matrix This drawback of direct reconstruction is commonly avoided by using a different reconstruction procedure. It is possible to enforce a physical, positive-semi-definite density matrix as an output, and to use a maximum likelihood estimation (MLE) procedure to find a density matrix that is most compatible with the experimental data [30] . Using numerical optimization, density matrices that form a best fit with the measurement results are sought. Such density matrices are properly normalized (have trace=1), are strictly non-negative and Hermitian, and can therefore be regarded as physical [30] (see Supplementary Note 3 ). 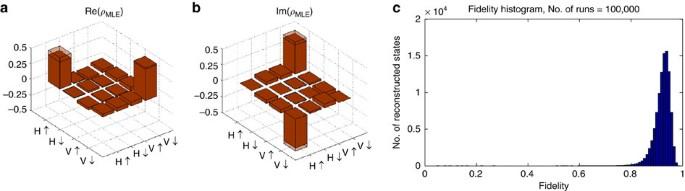Figure 3: Density matrix reconstruction through least-squares estimation. (a) Real part of the density matrix obtained using the MLE procedure described in the text. The ideal density matrix (ρideal) is overlayed (shaded box). (b) Imaginary part of the density matrix obtained using the MLE procedure described in the text. The ideal density matrix (ρideal) is overlayed (shaded box). (c) Histogram (100,000 runs) of the obtained fidelities using the MLE-reconstruction, taking into account the experimental uncertainties. The mean and median fidelities are over 92%, with standard errors of about 3.2%. Figure 3 shows the density matrix obtained from the MLE procedure. The fidelity is calculated using the same definition as for the direct reconstruction: . The non-zero measurement uncertainties (Poissonian counting statistics [21] ) imply that the fidelity of the reconstructed state will also have an uncertainty associated with it. To quantify this uncertainty, we calculated the MLE-reconstruction for a range of possible input measurements, randomly sampled from the distribution of the possible measurement results, using a Monte Carlo method—see Supplementary Note 3 . The resulting histogram (probability distribution) of the calculated fidelity is indicated in Fig. 3c , where 100,000 simulated noisy measurement results are used to calculate the MLE-obtained fidelity. We obtain a mean fidelity of 92.1% (median: 92.7%), with a standard deviation of 3.2%. The theoretical upper bound, determined by the timing resolution of the time-resolved conversion technique [21] , is around 95%, and is therefore close to being satisfied; residual errors in the pulse control of the spins account for most of the remaining difference (see Supplementary Note 1 ). Using the same methods, we calculated a concurrence of 0.908 (s.d. : 0.051), a tangle of 0.826 (s.d. : 0.086), an entanglement of formation of 0.87 (s.d. : 0.069) and a linear entropy of 0.107 (s.d. : 0.06). Figure 3: Density matrix reconstruction through least-squares estimation. ( a ) Real part of the density matrix obtained using the MLE procedure described in the text. The ideal density matrix ( ρ ideal ) is overlayed (shaded box). ( b ) Imaginary part of the density matrix obtained using the MLE procedure described in the text. The ideal density matrix ( ρ ideal ) is overlayed (shaded box). ( c ) Histogram (100,000 runs) of the obtained fidelities using the MLE-reconstruction, taking into account the experimental uncertainties. The mean and median fidelities are over 92%, with standard errors of about 3.2%. Full size image The entanglement fidelity becomes critically important if one intends to connect such multiple matter–light quantum interfaces to make a quantum repeater [7] , [8] . For each link in a repeater network, the photons from two spin–photon pairs interfere to produce a spin–spin Bell-state [16] , where the spin qubits are stored in separate repeater nodes at either end of the channel (see Fig. 4a ). The repeater node would have two or more photon-based interfaces to communication links and local quantum gates between spins and spin-state read-out in each repeater node transfer information through the network. To overcome errors, these local operations could also distil a high-fidelity Bell-state (say F ≥0.995) from multiple lower-fidelity pairs of entangled qubits [13] . 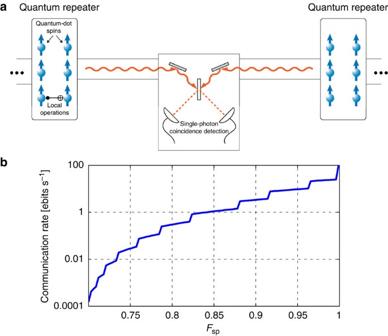Figure 4: Quantum dot spin–photon entangled pairs for quantum repeaters. (a) A schematic diagram of a quantum repeater based on optical quantum dots. When a spin–photon pair is generated, the spin is stored in the repeater node, whereas the photon is sent into the communication channel. Two such photons from different repeater nodes interfere to (probabilistically) produce spin–spin entanglement between two repeaters. (b) Plot of the simulated net communication rate of entangled spin–spin pairs after consumption (in purification) of ‘raw’ spin–photon states and EPR-Bell-pairs (Einstein-Podolsky-Rosen) suitable for use in the network. Entanglement distillation consumes many raw pairs generated atFss=+(1/3)(1−Fsp)2(assuming depolarizing noise). AsFspapproaches the threshold 0.71 from above, the net communication rate goes to zero. The communication rate in entangled bits per second (ebits s−1) is calculated, assuming spin–photon pairs interfering at a rate of 100 s−1. The final spin–spin entanglement fidelity is at least 0.995. Figure 4: Quantum dot spin–photon entangled pairs for quantum repeaters. ( a ) A schematic diagram of a quantum repeater based on optical quantum dots. When a spin–photon pair is generated, the spin is stored in the repeater node, whereas the photon is sent into the communication channel. Two such photons from different repeater nodes interfere to (probabilistically) produce spin–spin entanglement between two repeaters. ( b ) Plot of the simulated net communication rate of entangled spin–spin pairs after consumption (in purification) of ‘raw’ spin–photon states and EPR-Bell-pairs (Einstein-Podolsky-Rosen) suitable for use in the network. Entanglement distillation consumes many raw pairs generated at F ss = +(1/3)(1− F sp ) 2 (assuming depolarizing noise). As F sp approaches the threshold 0.71 from above, the net communication rate goes to zero. The communication rate in entangled bits per second (ebits s −1 ) is calculated, assuming spin–photon pairs interfering at a rate of 100 s −1 . The final spin–spin entanglement fidelity is at least 0.995. Full size image When two spin–photon pairs with fidelity F sp interfere, the resulting spin–spin entanglement fidelity F ss is lower-bounded by F ss ≥( F sp ) 2 , assuming perfect interference between the photons. Furthermore, it is known that entanglement distillation of EPR-Bell-states (Einstein-Podolsky-Rosen) has a ‘threshold’ lower bound of F ss >0.5 to increase fidelity at the output [13] . From this simple ansatz, we can draw two conclusions. First, and again assuming perfect photonic interference, using two spin–photon entangled pairs with measured fidelity F sp >1/ ≈0.71 will always result in a spin–spin entangled pair with fidelity F ss >0.5, which is above the threshold for purification. Conversely, for spin–photon fidelities below 0.71, it is not generally true that such a purifiable spin–spin entangled pair can be created. Although some lower-fidelity spin–photon states result in spin–spin entangled states that can be purified, more information about the particular state (via the knowledge of the full density matrix) would be required–see Supplementary Discussion . In this sense, 0.71 can be seen as an unconditional threshold for the spin–photon entanglement fidelity—a sufficient condition for scalability. To the best of our knowledge, this experiment is the first one in any solid-state system to unambiguously demonstrate (at the 99.9% confidence level) a spin–photon fidelity above this threshold. Second, and more importantly, the efficiency of entanglement distillation, which directly has an effect on the communication rate, increases as F sp →1. This effect can be seen clearly by the simulation results in Fig. 4b . Here we calculate the average net communication rate of high-fidelity ( F≥ 0.995) spin–spin entangled pairs by distillation from noisy spin–photon Bell states [8] . If one compares the performance of the two systems starting from F sp =0.9 versus F sp =0.8, the former has a higher communication rate by a factor of 10, illustrating the dramatic effect of improved spin–photon entanglement fidelity. For our experiment, the Monte Carlo uncertainty analysis used revealed that our spin–photon state has a fidelity above the threshold of 1/ with 99.9% certainty, and that our entangled state has a fidelity greater than 0.9 with 81.4% certainty ( Supplementary Table S1 ). In conclusion, we demonstrated a full tomographic analysis of high-fidelity spin–photon entanglement in a solid-state system using InAs quantum dots. The resulting fidelity would allow for efficient distillation of purified entangled states, and represents a milestone in the quest to build quantum networks. InAs quantum dot device We used a Si-δ-doped quantum dot (QD) sample, similar to previous devices [21] . The dot density was reduced, and the emission blue-shifted (910 nm). We obtained excellent collection efficiency by means of an asymmetric, low- Q cavity (10 nm full width at half maximum, centred at 910 nm) that reduces photon loss from the spontaneous emission into the substrate. An external magnetic field perpendicular to the growth direction (Voigt geometry) splits the electron spin states as well as the excited, trion states. Figure 1a indicates the resulting Λ-systems, and the polarization selection rules were verified by means of polarization-selective photoluminescence (half-waveplate and polarizing beamsplitter) [25] , [28] . We screened the device and selected those quantum dots with the cleanest selection rules, to suppress residual errors. Experimental setup A superconducting magnetic cryostat (Oxford Spectromag; the magnetic field used was varied between B =3 and 6 T) cooled the devices to a base temperature of 1.5 K. A 0.68-NA aspheric lens inside the cryostat focused the pump and rotation lasers onto the sample, which was scanned relative to the lens by means of slip-stick piezo-electric positioners (Attocube Systems). We used similar coherent manipulation techniques as those reported previously [25] . A narrowband continous-wave-laser (New Focus Velocity) was used for spin initialization and read-out, resonant to the - -transition (910.10 nm for a 3-T magnetic field); fibre-based electro-optic modulators (EOM, EOspace) were used to switch the laser light on and off. We used a Ramsey-interferometry setup for coherent spin rotations, using pulses from a modelocked laser (3 ps pulse duration, centre wavelength 911 nm, Spectra-Physics Tsunami), which were delayed relative to each other through a retroreflector on a motorized stage. Pulse-picking was realized using free-space EOMs (Conoptics), which were double-passed to increase the extinction ratio. The selective excitation of the -state prior to spontaneous emission was realized through a combination of optical pumping into the -state, rotation by an optical π -pulse into the -state, followed by the application of a 100-ps pulse (optical π -pulse) from another, synchronized, modelocked laser (Spectra-Physics Tsunami with Lok-to-Clock system), resonant with the - -transition. Pulse-picking of the 100-ps excitation pulses required another fibre-optic modulator. For the single-photon photoluminescence, we built a confocal setup, split into two branches by a non-polarizing beamsplitter. One branch was cross-polarized with respect to the initialization and optical pumping lasers, and sent through a double-monochromator onto a single-photon counter for spin-state analysis (Perkin-Elmer single-photon counting module; 20% quantum efficiency, 170 Hz ungated dark count rate). The other branch was sent to a polarization analysing stage (quarter- and half-waveplate and polarizer), after which it was coupled into single-mode fibres and sent to the downconversion setup. We carefully calibrated the polarization analysing stage, to account and compensate for residual birefringence in the setup. All EOMs were controlled by mutually synchronized pulse-pattern generators (76 MHz Tektronix and 10 GHz Anritsu PPG), themselves synchronized to the repetition rate of the modelocked lasers. Spatial, polarization, wavelength and time-filtering sufficed for separating reflected light from the single photons. Quantum erasure via frequency conversion For the 2.2-μm light pulses needed for conversion, we used a difference-frequency generation process that mixed the 3-ps, 911-nm pulses from the modelocked laser with narrowband, continous-wave 1560-nm light in an MgO-doped, PPLN chip. The 1560-nm light was modulated by a fibre-optic modulator, and amplified by erbium-doped fibre amplifiers. The residual 1560-nm and 911-nm light was filtered out through a combination of dichroic and absorptive filters. The resulting pulse width depended on the exact power and wavelength used for the difference-frequency generation process, but was measured to be between 3 and 8 ps. Conditional on exact temporal overlap, a PPLN waveguide efficiently converted 910-nm, spontaneously emitted photons to 1560-nm photons. To eliminate residual noise from the 910 nm and 2.2 μm branches, we installed a fibre-Bragg grating and a long-pass filter. The 1560-nm photons were subsequently detected on a superconducting nanowire single-photon detector, maintained at 2 K, with 14% system detection efficiency, 40-Hz ungated dark count rate and 100-ps full width at half maximum timing jitter. Timing analysis was performed on a timing analyser (Hydraharp, PicoQuant GmbH), used in time-tagged time-resolved mode, which allows for accurate gating of the signals of both the single-photon counting module and the superconducting nanowire single-photon detector in post-processing, thereby drastically reducing the effects of dark counts. The timing of the 2.2-μm light was chosen such that the subsequent π /2-pulse arrives after 70–100 ps, which is well within the -dephasing time of the quantum dot (1.5 ns), though spin-echo techniques could be used to overcome this limitation. Correlation analysis The correlation data that were used in the tomographic reconstruction algorithms, were the result of a histogram analysis, performed on the coincidence count rate between the downconverted single photons, and the single photons used for spin detection. The coincidence count rate was obtained through post-processing of the time-tagged time-resolved datastream, and comparing the coincidences within the same experimental run to those in subsequent, uncorrelated ones. The repetition rate is set at 39 or 52 ns, and the 0.1% single-photon efficiency and time-gated frequency downconversion resulted in a 1560-nm single-photon detection and entanglement generation rate of approximately 2–5 Hz. In combination with another 0.1% single-photon detection efficiency to detect the spin state (this efficiency is the result of all losses between the QD and the detector, including efficiency of collecting a photon from the QD into the optical path; losses from subsequent spatial, polarization and frequency filtering, finite detector quantum efficiency), this resulted in an average coincidence rate of approximately 2–5 mHz. We emphasize that these losses are predominantly due to the inefficiency of extracting a single photon from the quantum dot, which could be significantly improved by accurate cavity design. The conversion process in itself, although lossy due to the aggressive time-filtering to obtain good timing resolution, was rather effective, with internal quantum efficiencies estimated above 80%, and filtering losses of several dB maximum. How to cite this article: De Greve, K. et al. Complete tomography of a high-fidelity solid-state entangled spin–photon qubit pair. Nat. Commun. 4:2228 doi: 10.1038/ncomms3228 (2013).